The convergent evolution of defensive polyacetylenic fatty acid biosynthesis genes in soldier beetles The defensive and bioactive polyacetylenic fatty acid, 8 Z -dihydromatricaria acid, is sequestered within a wide range of organisms, including plants, fungi and soldier beetles. The 8 Z -dihydromatricaria acid is concentrated in the defence and accessory glands of soldier beetles to repel avian predators and protect eggs. In eukaryotes, acetylenic modifications of fatty acids are catalysed by acetylenases, which are desaturase-like enzymes that act on existing double bonds. Here we obtained acyl Coenzyme A-linked desaturases from soldier beetle RNA and functionally expressed them in yeast. We show that three genes were sufficient for the conversion of a common monounsaturated fatty acid, oleic acid, to the 18 carbon precursor of 8 Z -dihydromatricaria acid, that is, 9 Z ,16 Z -octadecadiene-12,14-diynoic acid. These are the first eukaryotic genes reported to produce conjugated polyacetylenic fatty acids. Phylogenetic analysis shows that the genes responsible for 8 Z -dihydromatricaria acid synthesis in soldier beetles evolved de novo and independently of the acetylenases of plants and fungi. More than 40 years ago, Meinwald et al . [1] reported the occurrence of a highly unusual fatty acid in the white viscous fluid released from exocrine defensive glands of the soldier beetle Chauliognathus lecontei Champion ( Cantharidae ). The compound was identified as 8 Z -dihydromatricaria acid (DHMA, Fig. 1 ) and was found to be a major component of the defensive secretion. The same acetylenic fatty acid was also discovered in the defence glands of the Australian soldier beetle, C. lugubris , along with a 12-carbon homologue as components of wax esters in female beetles [2] . Chauliognathus beetles are rejected by many potential vertebrate and invertebrate predators; Eisner et al . [3] demonstrated the potent anti-feedant activity of DHMA towards predatory spiders at dosages equivalent to those stored in a single defensive gland. DHMA and closely related compounds are widespread in plants, especially Solidago and Erigeron spp. daisies (family Asteraceae ), and in fungi, particularly among Basidiomycetes, for example, Polyporus anthracophilus [4] . Matricaria-type polyacetylenic fatty acids are unknown in animals other than Chauliognathus spp. soldier beetles. As soldier beetles have been observed to forage upon the flowers of the Asteraceae , and no other animals have been reported to contain DHMA, the presence of polyacetylenic fatty acids in these insects has been suggested to reflect dietary or other associations with DHMA-containing plants rather than de novo synthesis [5] , [6] . 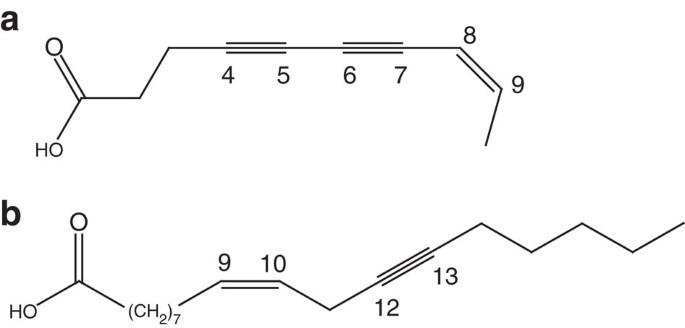Figure 1: Molecular structures of naturally occurring acetylenic fatty acids. (a) Dihydromatricaria acid and (b) Crepenynic acid (9Z-octadecene-12-ynoic acid). Figure 1: Molecular structures of naturally occurring acetylenic fatty acids. ( a ) Dihydromatricaria acid and ( b ) Crepenynic acid (9 Z -octadecene-12-ynoic acid). Full size image Recent progress has been made towards understanding the biosynthetic pathways of polyacetylenic fatty acids among terrestrial organisms. Members of the plant families Asteraceae , Apiaceae , Araliaceae and Solanaceae synthesize polyacetylenic fatty acid-related secondary metabolites that use crepenynic acid (9 Z -octadecene-12-ynoic acid, Fig. 1 ) as the precursor fatty acid. Divergent isoforms of the microsomal acyl lipid-linked fatty acid desaturases introduce an acetylenic bond into the Δ12 position of linoleic acid to form crepenynic acid in the daisy Crepis alpina [7] and in the chanterelle mushroom Cantharellus formosus [8] . However, to date, advancement of this field has been restricted to the first acetylenic bond formation in the Δ12 position and subsequent Δ14 unsaturation of the polyacetylenic biosynthesis pathway [8] . Fatty acid desaturases belong to a large family of non-heme diiron oxido-reduction enzymes that, in effect, remove two hydrogen atoms from adjacent carbons in a fatty acid chain to form a double bond, or in the case of acetylenases a further pair of hydrogens are removed from an existing double bond to produce a triple bond [7] , [9] . Integral-membrane desaturases are differentiated by their substrate preferences, either of the phospholipid-linked substrate preference found in plants and fungi, whereas acyl Coenzyme A (acyl-CoA)-linked preferences are mainly found in higher animals, including insects [10] , [11] . Aside from substrate preferences, the two groups of membrane desaturases also have very low gene and amino acid sequence identities. The challenging chemistry and variety of potent biological activities of polyacetylenic fatty acids, which includes activities against cancer cells, infecting microbes and plant alleopathy [12] , [13] , [14] , [15] , [16] , [17] , [18] , [19] , [20] , have excited interest among natural-product prospectors and bioactive discovery programmes, and have propelled our interest in new molecular structures and biosynthetic origins. In this report, we describe a three-gene pathway isolated from the Australian soldier beetle C. lugubris , leading to an 18-carbon precursor of DHMA, and the first eukaryote biosynthesis of conjugated polyacetylenic compounds. Further, we reveal that DHMA production in soldier beetles is likely to proceed via crepenynic acid as an intermediate, previously found only in plants and fungi, but its biosynthesis pathway has been convergently evolved to those of plants and fungi. Tissue analysis DHMA was confirmed in our analysis as the major polyacetylenic fatty acid in male adult Australian soldier beetles at <1% of total fatty acids, which is in accordance with a previous report [2] . However, extraction of tissue samples from mature female beetles and analysis of fatty acid methyl esters (FAMEs) by gas chromatography/mass spectrometry (GC/MS, electron ionization) gave a range of polyacetylenic fatty acids. DHMA was the major polyacetylenic fatty acid detected in eggs in situ , and almost 90% of total FAME from accessory glands was present as a C12 homologue of DHMA ( Supplementary Fig. S1 ). Cloning of the soldier beetle desaturases Eleven partial nucleic acid sequences, denoted CL1-11 , encoding likely desaturases were amplified from soldier beetle RNA using degenerate primers designed from the sequences of characterized insect desaturases, as described in Methods. The partial sequences were aligned with equivalent sequence fragments from genome-annotated desaturases from the flour beetle Tribolium castaneum in which acetylenic fatty acids are absent. Selected on the basis of sequence divergence from the desaturases of T. castaneum , full-length soldier beetle sequences were obtained for CL1 (JQ619626), CL3 (JQ619629), CL4 (JQ619630) and CL10 (JQ619631), using 5′- and 3′-rapid amplification of cDNA ends (RACE), or by a modified RACE reaction. Two closely related clones of the CL2 ( CL2-1 JQ619627 and CL2-2 JQ619628 ) gene were obtained from RNA pooled from a mixture of insects; their nucleotide and amino acid sequences had 98.9% and 99.4% identity, respectively. Full-length sequence of what was likely to be the conserved Δ9 desaturase ( CL11 , JQ619632) was also obtained. All encoded protein sequences were confirmed as desaturases, as they contained the eight conserved histidine residues that form the 'histidine boxes' that are essential for desaturase activity [21] , were of length between 327–354 amino acids and were aligned with the desaturases of mammals and insects that utilize CoA-linked substrates ( Supplementary Fig. S2 ). Characterization of soldier beetle desaturases in yeast All full-length C. lugubris desaturases were heterologously expressed in Saccharomyces cerevisiae , where they may utilize endogenous fatty acids such as oleic, stearic and palmitoleic acids. Alternatively, yeast expressing C. lugubris desaturases or a vector control were incubated with exogenously supplied fatty acids to investigate a single step of conversion by providing a precursor fatty acid or to increase the amount converted to product. Expression of desaturase CL10 gave rise to several new fatty acids in cellular lipids compared with yeast expressing the control vector as demonstrated by new peaks appearing in the gas chromatogram of extracted FAMEs ( Fig. 2 ). These were identified as linoleic acid (9 Z ,12 Z -octadecadienoic acid), palmitolinoleic acid (9 Z ,12 Z -hexadecadienoic acid), linolelaidic acid (9 Z ,12 E -octadecadienoic acid) and crepenynic acid ( Fig. 2a ; Supplementary Fig. S3 ). Their identification was based on a comparison of GC retention times and mass spectra with authentic standards, in particular crepenynic acid ( Figs 2 and 3 ). This result suggested that CL10 was a dual-function Δ12 desaturase/acetylenase utilizing oleic, palmitoleic and linoleic acids as substrates. Crepenynic acid production was increased by additional feeding of yeast expressing CL10 with linoleic acid, but was not essential as CL10 produces sufficient linoleic acid to support the conversion ( Supplementary Fig. S3 ). 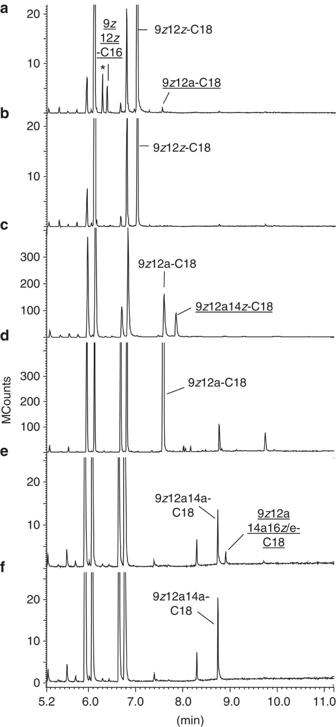Figure 2: Gas chromatograms of acetylenic products of soldier beetle genes expressed in yeast. Fatty acid methyl esters were prepared from yeast expressing soldier beetle desaturases (a) CL10 and (b) empty vector pYES2 provided with linoleic acid. (c) CL4 and (d) empty vector provided with crepenynic acid. (e) CL4 and (f) empty vector provided with 9z12a14a-C18. Yeast was supplied exogenously with 0.2 mM fatty acids and analysis was conducted using method 1. Key to fatty acids: 9z12z-C16 palmitolinoleic; 9z12z-C18 linoleic; 9z12a-C18 crepenynic; 9z12a14z-C18 dehydrocrepenynic; 9z12a14a-C18 9Z-octadecen-12,14-diynoic; 9z12a14a16z/e-C18 9Z,16Z/E-octadecadien-12,14-diynoic acid. Underlined fatty acids are new products. Chromatogramsaandbcorrespond to the ion current obtained by extraction of significant ions in the spectrum of methyl crepenynate—m/z79, 93, 236. Ina, the peak marked * eluting at 6.3 min was identified as 7Z,10Z-hexadecadienoic acid via analysis of the mass spectrum of the 4,4-dimethyloxazoline derivative and may arise from β-oxidation of linoleic acid (9z12z-C18) by yeast. Figure 2: Gas chromatograms of acetylenic products of soldier beetle genes expressed in yeast. Fatty acid methyl esters were prepared from yeast expressing soldier beetle desaturases ( a ) CL10 and ( b ) empty vector pYES2 provided with linoleic acid. ( c ) CL4 and ( d ) empty vector provided with crepenynic acid. ( e ) CL4 and ( f ) empty vector provided with 9 z 12a14a-C18. Yeast was supplied exogenously with 0.2 mM fatty acids and analysis was conducted using method 1. Key to fatty acids: 9 z 12 z -C16 palmitolinoleic; 9 z 12 z -C18 linoleic; 9 z 12a-C18 crepenynic; 9 z 12a14 z -C18 dehydrocrepenynic; 9 z 12a14a-C18 9 Z -octadecen-12,14-diynoic; 9 z 12a14a16 z /e-C18 9 Z ,16 Z / E -octadecadien-12,14-diynoic acid. Underlined fatty acids are new products. Chromatograms a and b correspond to the ion current obtained by extraction of significant ions in the spectrum of methyl crepenynate— m/z 79, 93, 236. In a , the peak marked * eluting at 6.3 min was identified as 7 Z ,10 Z -hexadecadienoic acid via analysis of the mass spectrum of the 4,4-dimethyloxazoline derivative and may arise from β-oxidation of linoleic acid (9 z 12 z -C18) by yeast. 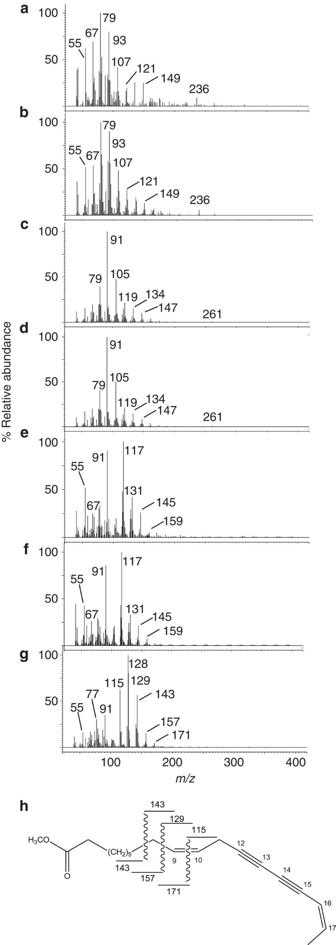Figure 3: Positive ion mass spectra of acetylenic fatty acid methyl esters. (a) 9z12a-C18 product of CL10 eluting at 7.57 min inFig. 2a, (b) pure standard of crepenynic acid; (c) 9z12a14z-C18 product of CL4 eluting at 7.8 min inFig. 2c,(d) pure standard of dehydrocrepenynic acid; (e) 9z12a14a-C18 product of CL2 eluting at 11.5 min inFig. 4a, and (f) pure standard of 9Z-octadecenedi-12,14-ynoic acid. (g) Putative 9Z,16Z-octadecadien-12,14-diynoic acid (9z12a14a16z/e-C18) eluting at 8.91 min inFig. 2eand (h) proposed mass spectral fragmentation pattern for the product. All mass spectra were acquired between 40–400 a.m.u. at 70 eV. Full size image Figure 3: Positive ion mass spectra of acetylenic fatty acid methyl esters. ( a ) 9 z 12a-C18 product of CL10 eluting at 7.57 min in Fig. 2a , ( b ) pure standard of crepenynic acid; ( c ) 9 z 12a14 z -C18 product of CL4 eluting at 7.8 min in Fig. 2c, ( d ) pure standard of dehydrocrepenynic acid; ( e ) 9 z 12a14a-C18 product of CL2 eluting at 11.5 min in Fig. 4a , and ( f ) pure standard of 9 Z -octadecenedi-12,14-ynoic acid. ( g ) Putative 9 Z ,16Z-octadecadien-12,14-diynoic acid (9 z 12a14a16 z /e-C18) eluting at 8.91 min in Fig. 2e and ( h ) proposed mass spectral fragmentation pattern for the product. All mass spectra were acquired between 40–400 a.m.u. at 70 eV. Full size image The activity of CL4 was highly specific and was restricted to introducing a double bond adjacent to an existing triple bond of two related substrates—crepenynic acid and 9 Z -octadecen-12,14-diynoic acid. The product of CL4 desaturation of crepenynic acid had the identical GC/MS characteristics as a standard of dehydrocrepenynic acid (9 Z ,14 Z -octadecadien-12-ynoic acid) extracted and purified from the chanterelle mushroom, Cantharellus cibarius ( Figs 2 and 3 ). In yeast expressing CL4, and supplied exogenously with 9 Z -octadecen-12,14-diynoic acid (prepared as described in Methods), the enzyme also exhibited Δ16 desaturase activity by producing 9 Z ,16Z-octadecadien-12,14-diynoic acid identified by examination of the mass spectrum and retention time of the product ( Figs 2 and 3g,h ). The two variants of CL2, CL2-1 and CL2-2, showed identical Δ14 acetylenase activity when expressed in yeast and fed exogenously with dehydrocrepenynic acid, which was converted to the conjugated diyne 9 Z -octadecen-12,14-diynoic acid ( Fig. 4a ). The identity of the latter was confirmed by matching the GC retention times and mass spectra of the product with the synthesized standard as shown in Figs 3d,e respectively. 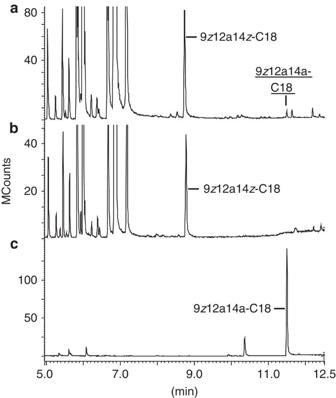Figure 4: Gas chromatogram of conjugated polyacetylenic fatty acid production by yeast expressingCL2. Fatty acid methyl esters were prepared from yeast expressing soldier beetle desaturases (a) CL2 and (b) pYES2 empty vector, supplied exogenously with 0.2 mM dehydrocrepenynic acid (9z12a14z-C18). (c) Synthesized standard (see Methods) of 9Z-octadecen-12,14-diynoic acid (9z12a14a-C18). Analysis was conducted using method 2. Figure 4: Gas chromatogram of conjugated polyacetylenic fatty acid production by yeast expressing CL2 . Fatty acid methyl esters were prepared from yeast expressing soldier beetle desaturases ( a ) CL2 and ( b ) pYES2 empty vector, supplied exogenously with 0.2 mM dehydrocrepenynic acid (9 z 12a14 z -C18). ( c ) Synthesized standard (see Methods) of 9 Z -octadecen-12,14-diynoic acid (9z12a14a-C18). Analysis was conducted using method 2. Full size image No other activities were observed for CL4 or 10 despite supplying yeast expressing the genes with a wide variety of fatty acid substrates, as listed in Supplementary Table S1 . An additional activity was observed for the CL2 variants; they converted exogeneously applied crepenynic acid to a small quantity of the methylene-interrupted diyne, octadeca-9,12-diynoic acid, and hence display Δ9 and Δ14 acetylenase activities. The activities of the remaining full-length desaturases determined through heterologous yeast expression were as follows: CL1 showed Δ12 desaturase activity towards oleic acid, producing a small quantity of linoleic acid (9 Z ,12 Z -octadecadienoic acid); CL3 had Δ9 desaturase activity exclusively toward myristic acid (tetradecanoic acid); and CL11 displayed high levels of Δ9 desaturation towards stearic and palmitic acids and is most likely the conserved Δ9 desaturase in the organism. Engineering of the polyacetylenic pathway in yeast Three C. lugubris genes, CL2-1 , CL2-4 and CL2-10 , were co-expressed in yeast to attempt the de novo production of polyacetylenic fatty acids. The products generated within the cells without exogenous supplementation were crepenynic and dehydrocrepenynic acids; the degree of substrate conversion to products are shown in Table 1 . Further acetylenase activity to form polyacetylenic fatty acids was detected only when additional dehydrocrepenynic acid substrate was supplied to yeast ( Table 1 ), indicating that this may be the rate-limiting step in the yeast model for the pathway. Table 1 Percentage conversion* of fatty acid substrates to products in yeast co-expressing soldier beetle CL2, CL4 and CL10 . Full size table Desaturase sequence relationships and phylogenetic analysis The encoded proteins of the full-length soldier beetle desaturase genes were most closely related to acyl-CoA Δ9 desaturases of the flour beetle, T. castaneum [22] , when subjected to BLASTP analysis against the non-redundant protein NCBI database. The Δ12 desaturase/acetylenase from C. lugubris (CL10) was found to be unrelated to Δ12 desaturase/acetylenases from the plant C. alpina or fungus C. formosus , as it had amino acid sequence identities of <12% with these sequences ( Supplementary Table S2 ). Furthermore, the Δ12 desaturase/acetylenase CL10 had low amino acid sequence identity to the insect Δ11/Δ13 desaturase/acetylenase isolated from the processionary moth ( Thaumetopoea pityocampa ; EF150363, ref. 23 ), and with Δ12 desaturases of T. castaneum (EU159449) and cricket Acheta domesticus (EU159448, ref. 24 ). An unrooted phylogenetic tree compiled from homeostatic, pheromone-, sex-specific and unknown function insect desaturases indicated that the soldier beetle desaturases and acetylenases involved in the biosynthetic pathway to polyacetylenic fatty acids (CL2, 4 and 10) form a well-supported clade together with other soldier beetle proteins, such as CL1, 3 and 11, and this clade was most closely related to the Δ9 desaturases of beetles ( Fig. 5 ). Notably, the soldier beetle desaturases were separated in the phylogenetic tree from Lepidopteran (moth) desaturases and acetylenases including the T. pityocampa Δ11/Δ13 desaturase/acetylenase, which lies among the Δ10–Δ13 desaturase/acetylenase sequences shown as a collapsed cluster in Fig. 5 . Because of the disproportionately large representation of moth desaturases, these sequences were collapsed into three main clusters in Fig. 5 to minimize the size of the tree, but were included, in full, in the analysis. 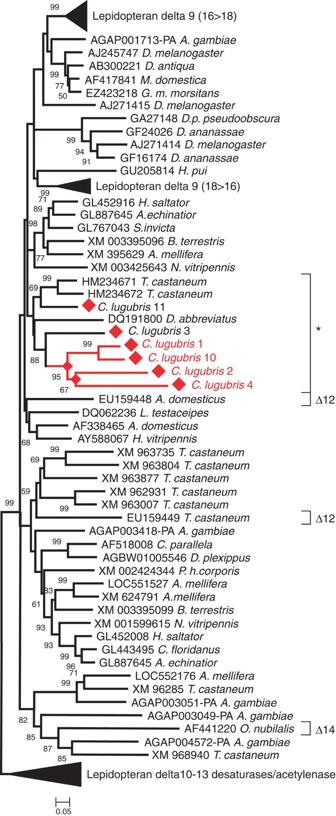Figure 5: Phylogenetic analysis of insect desaturases. A Neighbour-joining phylogenetic tree was prepared from all reviewed insect amino acid sequences held in Genbank. Statistical support for nodes with bootstrap values (resampling size of 1,000) are given at branch points, but only those with >50% support are indicated. Sequences are identified by Genbank nucleotide accession numbers, followed by an abbreviated genus and species name. Characterized activities of the desaturases (delta X; where X is the first point of unsaturation in the molecule, and numbers in parenthesis refer to the carbon chain-length specificity) are indicated at the right of the tree. The asterisked bracket indicates a clade of coleopteran (beetle) desaturases, including all full-length soldier beetle sequences (red diamonds) and those involved in polyacetylenic fatty acid formation (red branch lines). Figure 5: Phylogenetic analysis of insect desaturases. A Neighbour-joining phylogenetic tree was prepared from all reviewed insect amino acid sequences held in Genbank. Statistical support for nodes with bootstrap values (resampling size of 1,000) are given at branch points, but only those with >50% support are indicated. Sequences are identified by Genbank nucleotide accession numbers, followed by an abbreviated genus and species name. Characterized activities of the desaturases (delta X; where X is the first point of unsaturation in the molecule, and numbers in parenthesis refer to the carbon chain-length specificity) are indicated at the right of the tree. The asterisked bracket indicates a clade of coleopteran (beetle) desaturases, including all full-length soldier beetle sequences (red diamonds) and those involved in polyacetylenic fatty acid formation (red branch lines). Full size image The co-occurrence of DHMA as a major defensive chemical in both the flowers of some Asteraceae and defense glands of Chauliognathus spp. soldier beetles led some researchers to conclude that the insects sequester the plant-derived DHMA within their bodies rather than synthesize the chemical [5] , [6] . On the contrary, we have identified a three-gene biosynthesis pathway from the Australian soldier beetle, which, when examined as sequential steps, could convert oleic acid to an 18-carbon precursor of DHMA, 9 Z ,16 Z -octadecadien-12,14-diynoic acid, as shown in Fig. 6 . The activities of the 3 soldier beetle genes were restricted to 18-carbon chain-length substrates, and palmitoleic acid in the case of CL10 when tested against a wide range of exogenously supplied C10-C20 fatty acid substrates ( Supplementary Table S1 ). The clear molecular relationship of 9 Z ,16 Z -octadecadien-12,14-diynoic acid to DHMA, the chain-length specificity of the soldier beetle desaturases, together with our thorough accounting for all the expressed desaturases in the insect suggests CL2 , CL4 and CL10 are the genes responsible for DHMA synthesis in the soldier beetle. The biosynthesis of a 10-carbon polyacetylenic fatty alcohol from 18-carbon oleic acid was demonstrated in the fungi Tricholoma grammopodium to proceed via a crepenynic acid intermediate [25] and 18-carbon precursors were also proposed as the route of production of 10-carbon polyacetylenic fatty acids in the Asteraceae [26] . It appears that soldier beetles have adopted a similar biosynthesis pathway to the formation of DHMA. 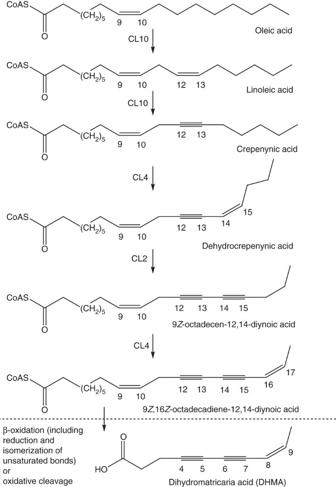Figure 6: Proposed dihydromatricaria acid biosynthesis pathway in soldier beetles. Scheme that shows the conversion of oleic acid to dihydromatricaria catalysed by three soldier beetle desaturases with subsequent chain shortening from C18 to C10 molecule via β-oxidation and reduction/isomerization, or via direct oxidative cleavage. Figure 6: Proposed dihydromatricaria acid biosynthesis pathway in soldier beetles. Scheme that shows the conversion of oleic acid to dihydromatricaria catalysed by three soldier beetle desaturases with subsequent chain shortening from C18 to C10 molecule via β-oxidation and reduction/isomerization, or via direct oxidative cleavage. Full size image The endpoint of the polyacetylenic fatty acid synthesis pathway described in Fig. 6 , 9Z,16Z-octadecadien-12,14-diynoic acid, was not identified in the dissected tissues of the soldier beetle. The product may undergo immediate chain shortening through targeted β-oxidation using normal unsaturated fatty acid degradation pathways, which include reduction and isomerization of unsaturated bonds, and then be stored within specific body tissues and glands. Alternatively, oxidation at carbon-9 and cleavage between carbon-8 and -9 could result in direct formation of 10-carbon polyacetylenic acids from 18-carbon precursors as reported in some plant species. Matricaria ester (methyl 2 Z ,8 Z -decene-4,6-diynoate) was detected in preparations of Matricaria trichophylla (Asteraceae) exposed to its 18-carbon precursor, or a precusor that included a ketone at carbon-9, with both substrates concluded to undergo oxidative cleavage between carbon-8 and -9 to form the short-chain ester [27] . Direct oxidative cleavage of 9 Z ,16 Z -octadecadien-12,14-diynoic acid to DHMA, if the pathway exists in soldier beetles, could explain the absence of 18-carbon or intermediate-length orthologues in insect tissues; however, a separate chain-shortening pathway would be needed to account for the presence of the C12 orthologue of DHMA. The enzymes involved in the formation of the 18-carbon DHMA precursor in soldier beetles were closely related to the acyl-CoA desaturases of mammals and other insects, enzymes that act on fatty acids to introduce unsaturated bonds in substrates linked to CoA. However, the soldier beetle Δ12 desaturase/acetylenase was only distantly related to another insect acetylenase, the multi-functional Δ11/Δ13 desaturase/acetylenase from the processionary moth, T. pityocampa [23] . Furthermore, sequence and phylogenetic analysis of the soldier beetle desaturases showed that the key proteins responsible for DHMA synthesis were most closely related to insect homeostatic Δ9 desaturases, from which they may have evolved, rather than more divergent forms. Indeed, the four proteins CL1, 2, 4 and 10 form a tight clade within the phylogenetic tree, suggesting a common ancestor for their evolution, which may have undergone multiple gene duplication events followed by changes of function through accumulated gene mutations [28] , [29] , [30] . The existence of a common ancestor is further supported by the desaturase sequences forming a discrete clade, despite each having developed divergent and distinctive catalytic activities. Crepenynic acid was a key intermediate in the soldier beetle biosynthetic pathway to polyacetylenic fatty acids and was formed by the action of a Δ12 acyl-CoA-type desaturase/acetylenase CL10 on linoleic acid. This is the first reported synthesis of crepenynic acid in animals; the genes conducting the identical transformation in the plant C. alpina and the chanterelle mushroom C. formosus have been identified [7] , [8] , but have essentially no sequence similarity to the soldier beetle Δ12 desaturase/acetylenase gene or encoded protein. In summarizing the evidence that soldier beetles have independently evolved a biosynthetic pathway to DHMA, to those of plants and fungi, we found a lack of sequence similarity between insect and plant/fungal Δ12 acetylenase proteins, but there was close relationship between the insect desaturases involved in homeostatic processes and those catalyzing formation of polyacetylenic fatty acids. Furthermore, the scarcity of defensive polyacetylenic fatty acids in insects indicates this biosynthetic pathway has arisen spontaneously within soldier beetles. Despite the likely separate evolution of the DHMA synthesis pathway in soldier beetles, it is possible that plant and fungal routes to DHMA and related fatty acids proceed via similar desaturase-catalysed steps; that is, following the formation of crepenynic acid, there is likely to be sequential formation of conjugated double and triple bonds on the 18-carbon fatty acid backbone, as we have reported for the synthesis by soldier beetle genes. Indeed, Blacklock et al . [8] have reported a fungal desaturase that acts on crepenynic acid to produce dehydrocrepenynic acid. Polyacetylenic fatty acids, containing more than one triple bond in the molecule, are produced and sequestered by a wide variety of organisms in many environments; more than 2,000 of these molecules have been identified in higher plants, liverworts, mosses, fungi, marine sponges and algae [19] . Many polyacetylenics have highly potent biological activities, which are used in defence against pathogens and predators [3] , [12] , [15] , and some have been investigated as human anti-cancer and anti-microbial treatments [13] , [16] , [18] , [20] . Conjugated polyacetylenic compounds are also very difficult to synthesize chemically; however, we have described a biosynthetic route using soldier beetle genes for heterologous production of these chemicals in yeast using mild conditions. More specifically, in this study we have discovered a eukaryotic gene and encoded protein (CL2) that catalyses the formation of conjugated diyne fatty acids, the key moiety for biologically active polyacetylenic compounds. Similar to its role in soldier beetles, DHMA and closely related compounds are considered defensive chemicals in members of the Asteraceae and in Basidiomycete fungi, and the molecule has certainly displayed a range of bioactivities in test batteries, including the following: anti-microbial activity [31] , as an anti-feedant [3] , depigmentation of melanocytes [32] , cytotoxicity [33] and ovicidal activity towards Drosophila melanogaster eggs [34] . The bioactive potency of DHMA is such that it has attracted the convergent evolution of its biosynthesis at least twice in evolutionary history—in soldier beetles and among plants/fungi. Extraction of beetle RNA and complementary DNA synthesis Adult male and female C. lugubris were collected from household gardens in Canberra, Australia, during summer and autumn (January–April). Adult beetles were dissected in PBS, and testis, fat body, defence glands, intestine, intestine-associated tissue, integument, eggs and egg sac, and female accessory glands were removed and separately extracted with 2:1 chloroform/methanol. The extracts were washed with saline and dried under a nitrogen stream, and FAMEs derivative of the lipids was prepared as described below. RNA was extracted from female and male beetles separately, or from mixed samples of C. lugubris (~100 mg) using the Trizol method following the manufacturers protocol (Invitrogen) or the RiboPure kit (Ambion Inc.; number AM1924). A yellow coloration remaining in the RNA was removed using the lithium chloride clean-up method from ToTALLY RNA (Ambion Inc.). First-strand cDNA was synthesized using the Invitrogen Superscript II kit. Purification of dehydrocrepenynic acid The methyl ester of dehydrocrepenynic acid was prepared from dried chanterelle mushroom, Cantharellus cibarius (La Tour Polignac Girolles Hanekammen), based on the method of Cahoon et al . [35] Methyl dehydrocrepenynate from chanterelle was verified by comparison of GC/MS retention time and mass spectra with a pure standard (Larodan, Sweden). Synthesis of 9 Z -octadecen-12,14-diynoic acid The -ene diynoic acid was prepared via copper coupling of methyl 11-bromo-9( Z )-undecenoate and 1,3-heptadiyne as detailed in the Supplementary Methods , and the resulting product was approximately 95% pure and matched the spectral characteristics with the product of a prior synthesis using a different approach [36] . The starting materials were prepared using the methods of Lie Ken Jie and Cheung [37] and Fiandanese et al . [38] , respectively. Cloning of soldier beetle desaturase sequences Degenerate PCR was performed using primers designed to conserved regions of insect desaturases as previously reported ( [24] ; Supplementary Table S3 ) and with an additional pair with sequence forward: 5′-GCNCAYMGNYTNTGGGCNCA-3′ and reverse: 5′-AANRYRTGRTGGTAGTTGIG-3′. The PCR cycling conditions were as follows: 94 °C for 3 min, and then 30 cycles of 94 °C for 15 s, 48 °C for 30 s, 72 °C for 2 min and then a final extension of 72 °C for 5 min. Amplification products of approximately 550 bp were excised and purified using the QIAgen PCR purification kit and cloned into pGEM T-Easy (Promega) vector system and sequenced. Full-length sequences of a soldier beetle desaturases were obtained by 5′- and 3′-RACE using the Clontech Creator SMART System, using gene-specific primers (GSPs; Supplementary Table S3 ). This gave full-length sequences for CL1 , CL3 , CL4 and two closely related sequences for CL2 . Full-length sequence of CL10 was obtained via a PCR-based method against a cDNA library generated from beetle RNA. GSPs ( CL10 GSP1: 5′-CCA AGC GTG GCT TCT TCT AC-3′; CL10 GSP2: 5′-CCC AGA AGT TTT CGG ATG AA-3′) were designed based on internal sequence data and used in combination with pDONOR 222 (Invitrogen) vector sequencing primers to amplify the 5′- and 3′-ends of the gene. The CL11 desaturase gene was amplified from genomic DNA using the Platinum Taq DNA Polymerase System (Invitrogen) and primers F2 and R2 [24] . Full-length sequence was obtained by 5′- and 3′-RACE using a 5′-RACE kit (Invitrogen), and GSP CL11F (5′- AAGCTT ATGGCTCCCAACATCTC-3′) and CL11R (5′- GGATCC TTAGAAAGATTTGACGT-3′) were used to amplify the desaturase from total RNA using the Superscript lll One-step RT–PCR System (Invitrogen). Functional characterization of C. lugubris desaturase genes Full-length C. lugubris desaturase genes were amplified by reverse-transcription PCR from total RNA for directional cloning into pYES2 (Invitrogen) using GSP ( Supplementary Table S3 ) and ligated into pGEM T-Easy (Promega), and the sequence was checked for correctness. Correct inserts were digested, gel-purified and ligated into pYES2 downstream of the GAL1 promoter and checked. Plasmids with soldier beetle desaturases were transformed into S. cerevisiae strains ole1 ( his3Δ1 , leu2Δ0 , ura3Δ0 , YMR272c::kanMX4 ) and INVSc 1 ( MATa , his3D1 leu2 trp1-289 ura3-52 ; Invitrogen). 10 Z -heptadecenoic acid (0.5 mM) and tergitol (NP-40; 1 %) were added in all media in which S. cerevisiae ole1 was grown. Transformants were selected on SCMM-U plates with 2% D -glucose. Functional characterization of C. lugubris desaturases was conducted in liquid culture, as described [22] , and in the presence of exogenously supplied fatty acids. After galactose addition to a final concentration of 2%, yeast cells were incubated in the presence of fatty acid substrates (final concentration 0.2 mM; Supplementary Table S1 ). FAME were prepared from yeast and accessory gland lipids using either sulphuric acid–methanol–chloroform or basic methoxide, and analysed by GC/MS as previously described [22] . Briefly, injections were made in the split mode using helium as the carrier gas, and the oven temperature was raised from 60 to 220 °C at 20 °C min −1 , then to 260 °C at 75 °C min −1 and held for 6.5 min (method 1) or alternatively from 60 to 180 °C at 20 °C min −1 , then 190 °C at 2.5 °C min −1 , then to 260 °C at 25 °C min −1 and held for 2.2 min (method 2). Co-expression of three C. lugubris desaturase gene pathway CL4 and CL2 were cloned into the pESC Trp yeast epitope tagging vector (Stratagene). CL2-1 was synthesized by Geneart AG (Germany) and subcloned into the Gal10 multiple cloning site. CL4 was amplified using GSP, purified and ligated into pGEM T-Easy (Promega). A verified CL4 sequence was subcloned into the pESC Trp Gal1 multiple cloning site using standard cloning methods. CL10 was cloned into the pYES2 vector and was co-transformed with pESC Trp containing CL2-1 and CL4 using the Yeast Transformation Kit (Sigma-Aldrich). Transformants were selected on SCMM-U, tryptophan with 2% D -glucose agar plates and sequence checked for appropriate gene inserts into the vectors. Sequence and phylogenetic analysis Phylogenetic analyses were conducted with insect desaturases having characterized activities, which included Δ9, Δ10, Δ11, Δ12, Δ13 and Δ14 desaturation, and uncharacterized proteins, alongside the sequences isolated from soldier beetle. We examined all putative insect desaturases held in Genbank and discarded truncated or otherwise incorrect sequences and closely related orthologues before alignment, using ClustalW with default parameters [39] . A phylogenetic tree was constructed with the Neighbour-joining method of Saitou and Nei [40] using the package MEGA4 (ref. 41 ). Bootstrap analysis with 1,000 replicates was carried out to determine statistical support for tree branches. How to cite this article: Haritos, V.S. et al . The convergent evolution of defensive polyacetylenic fatty acid biosynthesis genes in soldier beetles. Nat. Commun. 3:1150 doi: 10.1038/ncomms2147 (2012).